Proposed formation and dynamical signature of a chiral Bose liquid in an optical lattice Recent experiments on p -orbital atomic bosons have suggested the emergence of a spectacular ultracold superfluid with staggered orbital currents in optical lattices. This raises fundamental questions concerning the effects of thermal fluctuations as well as possible ways of directly observing such chiral order. Here we show via Monte Carlo simulations that thermal fluctuations destroy this superfluid in an unexpected two-step process, unveiling an intermediate normal phase with spontaneously broken time-reversal symmetry, dubbed a ‘chiral Bose liquid’. For integer fillings ( n ≥2) in the chiral Mott regime, thermal fluctuations are captured by an effective orbital Ising model, and Onsager’s powerful exact solution is adopted to determine the transition from this intermediate liquid to the para-orbital normal phase at high temperature. A lattice quench is designed to convert the staggered angular momentum, previously thought by experts difficult to directly probe, into coherent orbital oscillations, providing a time-resolved dynamical signature of chiral order. Orbital degrees of freedom and interactions play a crucial role in the emergence of many complex phases in solid state materials. High temperature superconductivity in the cuprates [1] and pnictides [2] , colossal magnetoresistance observed in Mn oxides [3] , and chiral p-wave superconductivity proposed in Sr 2 RuO 4 (ref. 4 ), are all nucleated by strong correlation effects in a multi-orbital setting [5] . For ultracold atomic gases, interaction effects combined with the band topology of p orbitals [6] have been argued to lead to exotic topological or superfluid (SF) phases for fermions [7] , [8] , [9] , [10] , [11] , [12] , [13] as well as bosons [14] , [15] , [16] , [17] , [18] , [19] , [20] , [21] , [22] , [23] , [24] , [25] . Interactions are predicted to drive a semi-metal to topological insulator quantum phase transition in two-dimensions (2D) for fermions in p x , p y and orbitals [12] , while interacting p -orbital atomic fermions in three-dimensions (3D) could lead to axial orbital order [26] . For weakly interacting 2D lattice bosons in p x and p y orbitals the ground state is proposed to be a SF with staggered p x ± ip y order [15] ; such order is also found for one-dimensional (1D) strongly interacting p -orbital bosons [24] . For bosons, these exotic phases can result from a particularly simple effect: repulsive contact interactions favour a maximization of the local angular momentum z , a bosonic variant of the atomic Hund’s rule for electrons [15] , [22] , [25] . Here we study p -orbital phases beyond their ground state properties, focusing on open fundamental issues such as thermal and dynamical effects, to be elaborated below. Our work is motivated by recent experiments that have successfully prepared long-lived metastable phases of weakly interacting 87 Rb atoms in p orbitals [21] , [27] . In the deep lattice regime, this experimental system is well approximated by a tight binding model on a checkerboard optical lattice with bosons in the p x , p y and s orbital degrees of freedom (see Fig. 1 ). The Hamiltonian of the model is obtained by extending the early theoretical studies [14] , [15] , [22] , [28] to the checkerboard lattice configuration used in the recent experiments of Wirth et al. [21] and Ölschläger et al. 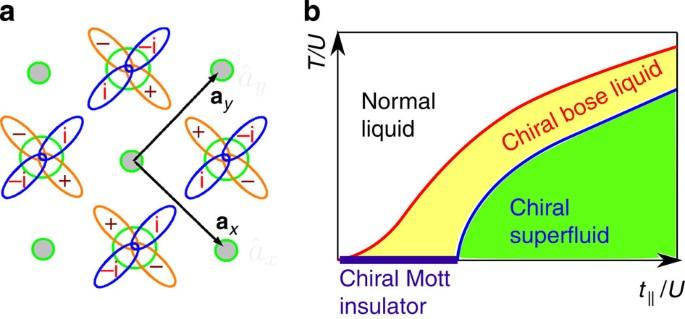Figure 1: Orbital lattice structure and phase diagram. (a) The checkerboard lattice structure as used in experiments to realizep-orbital superfluid21, together with the phases of the staggered orbital ordering in chiral states. The arrowsaxandayare primitive vectors of the square lattice. The symbols (+,i, −, −i) indicate the phases of each orbital wavefunction (0,π/2,π,3π/2), respectively. (b)The schematic phase diagram ofp-orbital band Bosons with fillingn≥2. The topology of the phase diagram is fixed by exact or controlled numerical and analytical calculations in the strong and weak coupling limits at non-zero temperature and for arbitrary coupling along theT=0 line of ‘Chiral Mott’ and is otherwise interpolated schematically elsewhere. At zero temperature there is a quantum phase transition between the chiral MI and superfluid phases, both of which break time-reversal symmetry. At finite temperature, there is a chiral Bose liquid phase. On heating, the chiral superfluid undergoes a BKT transition into the chiral Bose liquid, which subsequently undergoes an Ising transition at a higher temperature into a normal Bose liquid. [27] Restricting ourselves to nearest-neighbor tunnelling, the Hamiltonian is H = H tun + H loc , with tunnelling and local terms [27] , Figure 1: Orbital lattice structure and phase diagram. ( a ) The checkerboard lattice structure as used in experiments to realize p -orbital superfluid [21] , together with the phases of the staggered orbital ordering in chiral states. The arrows a x and a y are primitive vectors of the square lattice. The symbols (+, i , −, − i ) indicate the phases of each orbital wavefunction (0,π/2,π,3π/2), respectively. ( b )The schematic phase diagram of p -orbital band Bosons with filling n ≥2. The topology of the phase diagram is fixed by exact or controlled numerical and analytical calculations in the strong and weak coupling limits at non-zero temperature and for arbitrary coupling along the T =0 line of ‘Chiral Mott’ and is otherwise interpolated schematically elsewhere. At zero temperature there is a quantum phase transition between the chiral MI and superfluid phases, both of which break time-reversal symmetry. At finite temperature, there is a chiral Bose liquid phase. On heating, the chiral superfluid undergoes a BKT transition into the chiral Bose liquid, which subsequently undergoes an Ising transition at a higher temperature into a normal Bose liquid. Full size image Here, b x ( x ), b y ( x ) and b s ( x ) are bosonic annihilation operators of p x , p y and s orbitals at site x . The position vectors r = r x a x + r y a y , with integers r x and r y . The vector a x ( a y ) is the primitive vector of the square lattice in the x ( y ) direction ( Fig. 1 ). The positions of s orbitals are , , and . The density operators are defined as and . The angular momentum operator is Note that a square lattice C 4 rotational symmetry has been assumed. With an analysis of the time-of-flight momentum distribution, Wirth et al. [21] and Ölschläger et al. [27] found evidence suggesting a staggered p x ± ip y SF. However, a direct measurement of its key property—the angular momentum order—remains a challenge. This is especially crucial in the absence of SF coherence, since quantum or thermal fluctuations may kill superfluidity while preserving chiral angular momentum order. This issue is also relevant to chiral electronic fluids proposed to emerge in Sr 2 RuO 4 (refs 29 , 30 , 31 ), doped graphene [32] and the pseudogap state of high-temperature superconductors [33] , [34] , [35] . While previous work has focused on the ground state properties of such unconventional Bose SFs, there remain important outstanding issues to be addressed. First, how do thermal or quantum fluctuations, which are important in any experimental setting, melt these unconventional SF states? Second, which experiment can directly detect the spatially modulated angular momentum underlying these unusual quantum states? And finally, what can one learn from the time-resolved dynamics of such complex orbital states? This brings us to two central results responding to the above open questions. First, using classical Monte Carlo simulations of an effective model of interacting p x and p y bosons, we show that thermal fluctuations lead to a two-step melting of the staggered p x ± ip y SF ground state. Sandwiched between a lower temperature Berezinskii–Kosterlitz–Thouless (BKT) transition at which superfluidity is lost, and a higher temperature Ising transition at which time-reversal symmetry is restored, lies a ‘chiral Bose liquid’ with spontaneously broken time-reversal symmetry. In other words, it is a remarkable state of matter that is chiral but not SF. For large Hubbard repulsion at integer fillings, n ≥2, a strong coupling expansion yields Mott insulating states with staggered p x ± ip y order. As shown schematically in Fig. 1 , this opens up a wide window in the phase diagram where staggered angular momentum order persists even in the absence of superfluidity. Our work represents the first study of the finite temperature properties of staggered p x ± ip y chiral Bose fluids. Second, mapping the p x , p y orbitals onto an effective pseudospin-1/2 degree of freedom, we show that one can simulate the spin dynamics in magnetic solids by orbital dynamics of p -band bosons. Specifically, we numerically study a particular lattice quench, using time-dependent matrix product and Gutzwiller states, which is shown to convert the angular momentum order of such chiral fluids into time-dependent oscillations of the orbital population imbalance, analogous to Larmor spin precession. These oscillations directly reveal the experimentally hard-to-detect ‘hidden order’ associated with spontaneous time-reversal symmetry breaking. This quench is analogous to nuclear magnetic resonance schemes in liquids or solids, which tip the nuclear moment vector and study its subsequent precession using radio-frequency probes. This non-interferometric, and time-resolved, route to measuring the angular momentum order works in SF as well as non-SF regimes, and it could be implemented using recent experimental innovations [36] , [37] , [38] . Chiral Bose liquid and Mott insulator at strong coupling We begin with the strong coupling regime, where atoms can localize to form a Mott insulator (MI) ground state. When the s orbitals in one of the sublattices ( Fig. 1 ) are largely mismatched in energy with the p orbitals, with a gap Δ sp , the nearest-neighbor tunnelling Hamiltonian for bosons dominantly residing in the p orbitals is given by with hopping amplitudes being mediated by the s orbitals. At integer filling, with n ≥2, a strong p -orbital Hubbard repulsion in equation (2) favors a local state with a fixed particle number with non-zero angular momentum in order to minimize the interaction energy [22] , [24] , [25] , [28] , leading to a MI with a two-fold degeneracy of orbital states p x ± ip y at each site. This extensive degeneracy is lifted by virtual boson fluctuations within second order perturbation theory in the boson hopping amplitudes. This effect is captured, by setting z ( r )= σ z ( r )| z ( r )|, and deriving an effective exchange Hamiltonian between the Ising degrees of freedom σ z ( r ), where . The chiral MI ground state thus supports a staggered (antiferromagnetic) angular momentum pattern, with a non-zero order parameter out to arbitrarily strong coupling. Such staggered time-reversal symmetry broken MIs, albeit for far more delicate plaquette currents, are known to emerge in frustrated Bose Hubbard models without orbital degrees of freedom, but only in an extremely small parameter window of interactions [39] , [40] , [41] . As schematically shown in Fig. 1 , heating this MI leads to a ‘chiral Bose liquid’ with spontaneously broken time-reversal symmetry. It only reverts to a conventional normal fluid above a symmetry restoring thermal phase transition of , which occurs at k B T I ≈2.27 adopted from the exact result [42] . Taking =0.02 and U =1 in units of the recoil energy of the optical lattice, we estimate the Ising transition temperature in the experimental system [21] , [27] to be ~1nK, well within the reach of cooling techniques in optical lattices. Monte Carlo simulations at weak coupling At low temperature, and with decreasing interaction strength, we expect both the chiral Bose liquid and the chiral MI to become unstable to superfluidity [25] . Equivalently, decreasing temperature at weak coupling is expected to lead to a sequence of transitions from normal to chiral Bose liquid and subsequently to chiral SF as shown in Fig. 1b . To address this physics in the weak coupling limit, we begin with the Hamiltonian , supplemented with local p -orbital interactions For small , the band structure of p -band bosons has minima at (π, 0) and (0, π). Interactions scatter boson pairs from one minimum into the other, leading the bosons to condense into a superposition state of the two modes, phase-locked with a relative phase ±π/2. This gives rise to a p x ± ip y SF ground state with a spontaneously broken time-reversal symmetry and non-zero staggered angular momentum order. To study the impact of thermal fluctuations on this weakly correlated SF, we make the reasonable assumption that classical phase fluctuations dominate the universal physics in the vicinity of the thermal phase transitions of this SF. This allows us to ignore the subdominant density fluctuations, and to replace , with ρ being the boson density, arriving at an effective classical phase-only Hamiltonian where Δ j θ α ( r )= θ α ( r + a j )– θ α ( r ) with j = x , y , and U ≈ ρ 2 U p /6. A more powerful symmetry-based effective field theory (EFT) approach (see Methods) confirms exactly the same lattice-regularized model. Using Monte Carlo simulations (see Methods), we have studied the thermal phase diagram of this model for fixed U / , with =1. As shown in Fig. 2a , the Binder cumulant [43] B L ( z ) for the staggered angular momentum order, computed for U / =1 on L × L systems with various L , exhibits a unique crossing point at T / =2.088(3), signalling a critical point with a diverging correlation length. The critical value of this Binder cumulant is B *≈0.61, very close to the universal 2D Ising value ≈0.61069 for the aspect ratio of unity and periodic boundary conditions used in our simulations. This suggests that the staggered angular momentum order disappears at T I / =2.088(3) via a thermal transition in the 2D Ising universality class. We confirm this from the scaling collapse of the order parameter curves shown in Fig. 2b using 2D Ising exponents ν =1 and β =1/8. 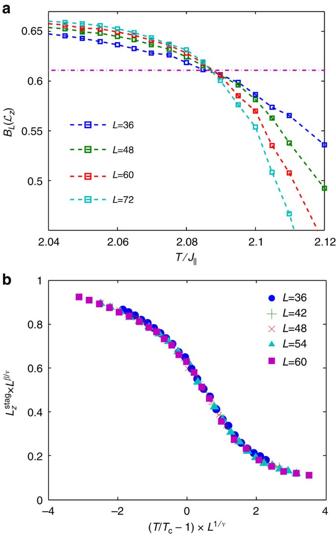Figure 2: Monte Carlo simulation for the angular momentum ordering of thepx±ipysuperfluid. (a) Binder cumulantBL(z) of the staggered angular momentum order parameter for different system sizesLshowing a crossing point at the Ising transition atT/=2.088(3). The dash dotted line indicates the universal value of the critical Binder cumulant 0.61069… for a 2D Ising transition. (b) Scaling collapse of the angular momentum order parameter curves for Ising exponentsν=1 andβ=1/8. Figure 2: Monte Carlo simulation for the angular momentum ordering of the p x ± ip y superfluid. ( a ) Binder cumulant B L ( z ) of the staggered angular momentum order parameter for different system sizes L showing a crossing point at the Ising transition at T / =2.088(3). The dash dotted line indicates the universal value of the critical Binder cumulant 0.61069… for a 2D Ising transition. ( b ) Scaling collapse of the angular momentum order parameter curves for Ising exponents ν =1 and β =1/8. Full size image To track the destruction of superfluidity, we have computed the atom momentum distribution function , which is accessible via time-of-flight measurements, as well as the SF stiffness ρ s (see Methods). On general grounds, a 2D quasi-condensed SF is expected to lose its superfluidity via a BKT transition driven by vortex unbinding, and it has been observed in trapped ultracold atom SFs. The BKT transition is signalled by a jump in ρ s satisfying the universal relation ρ s ( T BKT )=2 T BKT /π. As seen from Fig. 3a , ρ s indeed appears to have a sharp drop in the temperature range 2.05–2.10, rounded by finite size effects. To confirm the BKT nature of the SF transition, and to precisely locate T BKT , we resort to three distinct approaches. The first uses the finite-size scaling of ρ s . Weber and Minnhagen [44] have derived the finite-size scaling of the SF density at T BKT . An unbiased fit to this log-scaling form (see Methods) shows that the fit error ( Fig. 3c ) exhibits the expected deep minimum at the BKT transition, enabling us to estimate T BKT / =2.072(3), and ρ s ( T BKT )/ T BKT ≈0.64. The latter is close to the universal value 2/π=0.6366…, providing further concrete evidence of a BKT transition. The second uses finite-size scaling of the transition temperature. We identify the finite-size BKT transition temperature T c ( L ) via ρ s ( T c ( L ), L )=2 T c ( L )/π. Above a BKT transition, the correlation length , yielding a finite-size scaling form ( σ and L 0 are non-universal numbers). An extrapolation using this formula, as shown in Fig. 3b,d , yields T BKT / =2.065(4). The third uses the momentum distribution n ( k ). As shown in Fig. 3e , n ( k ) exhibits equal height peaks at k 1 =(π, 0) and k 2 =(0, π). This is consistent with the weak coupling analysis, which shows degenerate p -band dispersion minima at these momenta. At a BKT transition, n ( k i ) ∝ L 7/4 (in contrast to scaling as ρ c L 2 for a true Bose condensate with a condensate density ρ c ). This implies that the scaled momentum distribution n ( k i ) L −7/4 should cross at T BKT for varying system sizes L . The plot of this scaled distribution ( Fig. 3f ) indeed reveals a unique crossing point, which yields T BKT / ≈2.067(3). 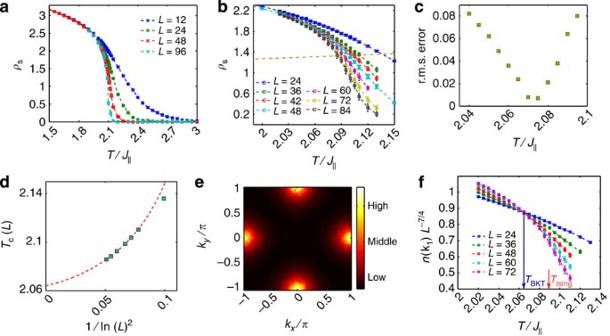Figure 3: Monte Carlo simulation for the superfluidity ofp-orbital bosons. (a) The superfluid stiffnessρsplotted over a wide range of temperature showing a rapid drop consistent with finite size effects at a BKT transition. (b)ρsfor a wide range of system sizes near the transition. (c) The r.m.s. error from fittingρs(L) to the Weber–Minnhagen log-scaling form at different temperatures with a steep minimum at the BKT transition pointT/=2.072(3). The dash dotted line in (b) shows 2T/π and its crossing with the curvesρs(T) defines finite size BKT transition temperatures, obeying a scaling relationTc(L)=TBKT+σ/ln2(L/L0) (see text). The extrapolation ofTc(L) to the thermodynamic limit shown in (d) predictsTBKT/=2.065(4). (e) Momentum distribution over the Brillouin zone, with equal height peaks atk1≡(π,0) andk2≡(0,π). (f) Scaled momentum distributionn(k1)L−7/4for different system sizesL, showing a crossing at 2.067(3), the BKT transition point. Also shown is the Ising transition temperature determined previously from the Binder cumulant analysis. Stated error bars on the transition points include statistical as well as extrapolation errors where applicable. Figure 3: Monte Carlo simulation for the superfluidity of p -orbital bosons. ( a ) The superfluid stiffness ρ s plotted over a wide range of temperature showing a rapid drop consistent with finite size effects at a BKT transition. ( b ) ρ s for a wide range of system sizes near the transition. ( c ) The r.m.s. error from fitting ρ s ( L ) to the Weber–Minnhagen log-scaling form at different temperatures with a steep minimum at the BKT transition point T / =2.072(3). The dash dotted line in ( b ) shows 2 T /π and its crossing with the curves ρ s ( T ) defines finite size BKT transition temperatures, obeying a scaling relation T c ( L )= T BKT +σ/ln 2 ( L / L 0 ) (see text). The extrapolation of T c ( L ) to the thermodynamic limit shown in ( d ) predicts T BKT / =2.065(4). ( e ) Momentum distribution over the Brillouin zone, with equal height peaks at k 1 ≡(π,0) and k 2 ≡(0,π). ( f ) Scaled momentum distribution n (k 1 ) L −7/4 for different system sizes L , showing a crossing at 2.067(3), the BKT transition point. Also shown is the Ising transition temperature determined previously from the Binder cumulant analysis. Stated error bars on the transition points include statistical as well as extrapolation errors where applicable. Full size image All three methods to locate T BKT yield consistent answers. Combining these results, our best estimate for the SF transition temperature is T BKT / ≈2.069(4). For = U =0.3, in units of recoil energy of the experimental optical lattice [21] , [27] , we estimate T BKT ~50 nK. Our numerical study unambiguously shows that the chiral p x ± ip y SF undergoes a two-step destruction: a lower temperature BKT transition at which superfluidity is lost, followed by a higher temperature Ising transition at which time-reversal symmetry is restored, leading to an unconventional ‘chiral Bose liquid’ at intermediate temperatures 2.069(4) ≲ T / ≲ 2.088(3). Such multiple transitions are also proposed to be relevant for 2D spinor condensates [45] . With increasing correlations, the BKT transition temperature is expected to get suppressed, eventually vanishing at the Mott transition (for integer fillings n ≥2), while the Ising transition remains non-zero for arbitrarily large repulsion as seen from our strong coupling results. Correlation effects thus enhance the window where one realizes a ‘chiral Bose liquid’ as shown in the schematic temperature-interaction phase diagram in Fig. 1 . Quantum quench and single-site orbital dynamics One can draw a fruitful analogy between the two orbital states at each site p x , p y and a pseudospin-1/2 degree of freedom ↑,↓. This suggests that one can simulate spin dynamics in solid state materials by studying orbital dynamics of p -band bosons. As we will see, this also suggests a route to directly detecting the angular momentum order in the p x ± ip y SF and ‘chiral Bose liquid’ of the type we have obtained. In our analogy, the p x ± ip y state corresponds to a pseudospin pointing along the y direction in spin space. Applying a ‘magnetic field’ along the x direction to this pseudospin should then induce Larmor precession, leading to periodic oscillations of the z -magnetization, corresponding to oscillations in the orbital population imbalance N ( p x )– N ( p y ). Let us imagine we prepare the system in a certain initial state, and then suddenly quench to a state where we set U p = U s =0, turn off all hoppings so t =0, and turn on a ‘magnetic field’ term at time τ =0; we later discuss how to realize such a term in optical lattice experiments. The staggered sign leads to a staggered coupling between the p x and p y orbitals. If initially a staggered superposition p x ± e i θ p y is prepared, this results in a rectification of all local Larmor precessions such that they add up to produce a macroscopic oscillation of the populations of the p x and p y orbitals. The p -orbital imbalance, , evolves, within a Heisenberg picture, as where is the staggered angular momentum operator whose evolution is in turn given by This leads to periodic oscillations of Δ N ( r ,τ)=‹Δ N ( r ,τ)› as where Δ N ( r , 0) and ( r , 0) denote the initial orbital magnetization and staggered angular momentum, respectively. Neglecting possible spatial inhomogeneity in λ ( r ) and φ ( r ), by focusing at the trap centre, we can set λ ( r )= λ and φ ( r )= φ , and extract the initial angular momentum order from the amplitude A ( r ) and the phase shift φ in the dynamics of the averaged number difference with N s being the number of lattice sites at the trap centre, and denoting the spatial average of (…). The coefficient λ can be directly read-off from the oscillation period τ Q ≡ π/ λ . We emphasize here that suitably averaged over the entire trap can be measured in time-of-flight experiments [21] . For a state with non-zero staggered angular momentum order, but no initial orbital population imbalance, that is, Δ N ( r ,0)=0, such as our chiral fluids, we expect ( τ ) to oscillate with a non-zero amplitude, and a phase shift φ =±π/2 whose sign will fluctuate from realization to realization, reflecting the spontaneous nature of time-reversal symmetry breaking. The amplitude of the signal will then be a direct measure of the staggered angular momentum order parameter, vanishing in a singular manner at the Ising phase transition, which restores time-reversal symmetry. In contrast, a completely thermally disordered conventional normal fluid would have ( τ )=0. A state with an initial orbital population imbalance but no angular momentum order, obtained by explicitly breaking the square lattice C 4 symmetry in the initial Hamiltonian as achieved in recent experiments, would exhibit oscillations with a nonsingular amplitude and a phase shift φ =0. Finally, if spontaneous time-reversal symmetry breaking exists in a system without C 4 symmetry, the amplitude of ( τ ) will be nonsingular while its phase shift will change in a singular manner, going from φ =±π/2 in a completely ordered state to φ =0 at the time-reversal symmetry restoring phase transition. Since this quench induced orbital magnetization dynamics is inherently a non-interferometric probe of the angular momentum order, it suggests a simple and powerful method for measuring time-reversal symmetry breaking in SF as well as non-SF chiral states. Our proposal thus significantly extends the earlier proposed quench dynamics approach for probing generic current orders [46] , [47] . In the presence of SF order, our real space quench is analogous to the recent proposal of Cai et al. [48] , which proposes to extract the relative phase between the p x and p y orbitals by studying momentum spectra after applying a Raman pulse to the Bose condensate. However, our proposal differs in showing that the angular momentum order can be probed irrespective of long range phase coherence or sharp momentum peaks. Numerical simulations of quench dynamics Our above analysis assumed that the quantum quench was complete, that is, all tunnelings ( t ) and interactions ( U ) were entirely switched off when H mag was switched on. We now show, using numerical simulations, that the coherent orbital oscillations are robust even with small non-zero tunnelings and interactions present after the quench, that is, for an incomplete quench. Since the scheme we are proposing here directly measures the local angular momentum order, it does not rely on the system dimensionality (beyond the assumption of long-range order). We therefore numerically simulate the zero temperature quench dynamics of a 1D model of p -orbital bosons, using both time-dependent Gutzwiller mean field theory [49] and time-dependent matrix product states (tMPS), finding good agreement at both weak and strong couplings and qualitatively similar conclusions at intermediate interaction strength. We then use the Gutzwiller mean field theory to also simulate the dynamics for the 2D case relevant to current experiments. The Hamiltonian of the 1D system is [24] where j index lattice sites. The ground state phase diagram of this 1D system includes two types of Mott states at strong coupling: a chiral Mott with staggered angular momentum order, and a non-chiral MI. For weak correlations, it supports two types of SF ground states: a chiral SF with staggered angular momentum order and a non-chiral SF [24] . The chiral states have an order parameter , with , which is analogous to the 2D case. We start with different ground states of H 1D and study their time evolution under a quantum quench that suddenly changes the Hamiltonian to H 1D +Δ H 1D , where The oscillatory dynamics of and is confirmed even for these entangled many-body states ( Fig. 4 ). Since the 1D geometry does not possess C 4 symmetry, we expect the different states to be distinguished by the phase shift φ , not the amplitude, of the oscillatory dynamics. The chiral Mott and SF states develop a periodic motion with non-zero phase shift. The dynamics of non-chiral states indicate zero phase shift. In this way the chiral states can be distinguished from non-chiral states by measuring the phase shift, which is directly related to the angular momentum order parameter. Deep in the chiral SF state, the phase shift is φ =±π/2, and it decreases in magnitude on approaching the chiral–non-chiral critical point. The phase shift vanishes in a singular fashion at this quantum critical point, signalling that this phase transition associated with time-reversal symmetry can be probed by measuring the order parameter via the phase shift φ . 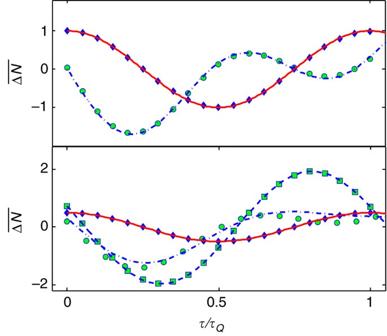Figure 4: Quench dynamics of 1D phases. Dots and lines are results of tMPS and Gutzwiller methods, respectively. The upper (bottom) panel shows dynamics of Mott (superfluid) states. In the upper panel the dash dotted line with circles and the solid line with diamonds correspond to chiral (two particles per site) and non-chiral (one particle per site) Mott states, respectively. In the bottom panel, the dash dotted line with circles and the dashed line with squares correspond to two chiral superfluid states with filling at 1.5 and 2, respectively; the solid line with diamonds is for a non-chiral superfluid state with filling at 0.5. For the chiral superfluid state with filling at 2,=U/3=λ/10 is used, and for the other states=0.045U=0.09λis used. The time unitτQis π/λ. Figure 4: Quench dynamics of 1D phases. Dots and lines are results of tMPS and Gutzwiller methods, respectively. The upper (bottom) panel shows dynamics of Mott (superfluid) states. In the upper panel the dash dotted line with circles and the solid line with diamonds correspond to chiral (two particles per site) and non-chiral (one particle per site) Mott states, respectively. In the bottom panel, the dash dotted line with circles and the dashed line with squares correspond to two chiral superfluid states with filling at 1.5 and 2, respectively; the solid line with diamonds is for a non-chiral superfluid state with filling at 0.5. For the chiral superfluid state with filling at 2, = U /3= λ /10 is used, and for the other states =0.045 U =0.09 λ is used. The time unit τ Q is π/ λ . Full size image Comparing time-dependent Gutzwiller [50] and tMPS methods ( Fig. 4 ), we find that the Gutzwiller approach captures orbital dynamics fairly well. We thus apply this approach to study orbital dynamics of the 2D system, as in experiments [21] . We have verified that a partial quench leads to long-lived Δ N oscillations as long as t and U are weak compared with the quench strength, that is, and . These results are shown in Fig. 5 . 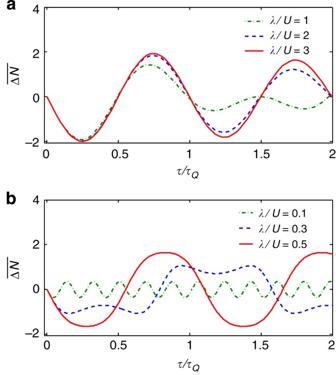Figure 5: Quench dynamics of 2D phases with various quench strengths via Gutzwiller approach. (a) and (b) show the evolution of ΔNfor chiral Mott states (with=0.0125Up) and superfluid states (=Up), respectively. The filling is ‹n(r)›=2. The time unitτQis π/λ. Non-chiral phases (not shown) have ΔN=0, and do not exhibit any post-quench oscillations. Figure 5: Quench dynamics of 2D phases with various quench strengths via Gutzwiller approach. ( a ) and ( b ) show the evolution of Δ N for chiral Mott states (with =0.0125 U p ) and superfluid states ( = U p ), respectively. The filling is ‹ n ( r )›=2. The time unit τ Q is π/ λ . Non-chiral phases (not shown) have Δ N =0, and do not exhibit any post-quench oscillations. Full size image Experimental proposal for quench To engineer the Hamiltonian H mag of Equation (8), we implement a quench potential V mag ( x ) modulated in the (1,1) direction in addition to the lattice potential giving rise to the quench Hamiltonian with which is valid in the tight binding regime when the quench potential is weak as compared with the original optical lattice (see Supplementary Note 1 ). Here, ω 0 is the harmonic oscillator frequency of the lattice wells hosting the p orbitals, and a ≡| a x |=| a y | is the lattice constant. Since the local density operator of the p orbitals n p ( r ) commutes with Δ N ( r ) and , it does not contribute to the dynamics of Δ N ( r ), and hence may be neglected. This is verified in our Gutzwiller simulations. We choose the quench potential as with some integer ν ≥0, a positive amplitude Γ, and K x , K y denoting the primitive vectors of the reciprocal lattice ( a i · K j =2πδ ij with i , j ε{ x , y }). The quench potential provides a lattice along the (1,1) direction, and it breaks both C 4 symmetry and mirror symmetries in the x and y directions. The potential is minimal at every second site of the Bravais lattice at positions r (= r x a x + r y a y ) with even r x + r y and it is maximal for all adjacent sites specified by odd r x + r y . Hence, the second derivative in Equation (15) produces the alternating sign required for realization of the quench Hamiltonian in Equation (8). Combining Equations (16) and (15) yields with E rec ≡ ħ 2 k 2 /2 m denoting the single photon recoil energy for photons with wave number . The lattice potential together with the corresponding quench potential can be realized by superlattice techniques demonstrated in several experiments [20] , [21] , [36] , [51] . For example, following Wirth et al. [21] , the lattice potential arises via two optical standing waves oriented along the (1,1) and (1,−1) axes with a wave number =2π/1,064 nm. The corresponding quench lattice requires an additional standing wave along the (1,1) axis with wave number . Hence, the case ν =1 requires ≈2π/709 nm, which is experimentally readily provided by diode laser sources. Both standing waves along the (1, 1)-direction may be derived by retro-reflecting two parallelly propagating laser beams with wave numbers k and k ′ by the same mirror. To prepare the required spatial relative phase of the two lattices, k ′ may be slightly detuned from the precise ratio k ′/ k = In most cold atom experiments, the trap potential can induce a slowly varying inhomogeneity in the ‘magnetic field’ λ as δλ =max{ λ ( r )}–min{ λ ( r )}. We expect the oscillations of the trap averaged number difference to decay over a time-scale . Finally we emphasize that besides the angular momentum order parameter, the quantum quench proposal and a subsequent study of Δ N ( r , τ) using in-situ microscopy can also yield correlation functions of ( r ), from which the diverging correlation length near the transition from chiral Bose liquid to normal can be extracted. Monte Carlo simulations We carry out the Monte Carlo study of the Hamiltonian in Equation (7) using a Metropolis sampling of the phase configurations { θ x ( r ), θ y ( r )}, with 10 7 sweeps to equilibrate the system at each temperature, and averaging all observables over 10 8 configurations. To study the chiral order, we construct the angular momentum order parameter and compute its Binder cumulant [43] . The universal order parameter distribution at renormalization group fixed points leads to universal values of L →∞ ; on finite size systems, this yields Binder cumulant curves, which cross at the critical point associated with angular momentum ordering. The critical value B * of the Binder cumulant is well-known to be universal, independent of lattice structure and details of the Hamiltonian, and depending only on the aspect ratio and boundary conditions used in the simulations. For periodic boundary conditions on L × L lattices, B *≈0.61069 for the 2D Ising universality class. The SF stiffness ρ s is defined as the change in the free energy density in response to a boundary condition twist; for , it is explicitly given by where ‹ ⋯ › refers to the thermal average. At a BKT transition, ρ s ( T ) jumps to zero, with ρ s ( T BKT )/ T BKT =2/π, a universal value. On finite size systems, the universal SF stiffness jump gets severely rounded, and a careful finite-size scaling is required to extract T BKT . On the basis of the KT renormalization group equations, Weber and Minnhagen have shown [44] that ρ s ( T BKT , L ) scales as where c is a non-universal number. It is well-known that fitting to this log-scaling form at different temperatures leads to an error, which exhibits a steep minimum at T BKT , enabling us to extract T BKT from our simulations. An unbiased fit to ρ s ( T )/ T , using a two-parameter scaling form, further confirms the universal jump at the T BKT identified by the error minimum. Using this, we find k ≈0.64 from our simulations, in very good agreement with the KT value 2/π=0.6366.... Effective field theory description We now show that the Monte Carlo study in the Results section is a lattice model simulation of the EFT for weakly interacting bosons in the experiments [21] , which does not rely on tight binding approximation. In the band structure calculation for the lattice rotation symmetric case [21] , dispersion of the relevant p -band E p ( k ) has two degenerate minima at Q x =(π,0) and Q y =(0,π), around which low energy modes can be excited due to quantum and thermal fluctuations. This leads to a two-component EFT, where the fields are introduced as with Λ a momentum cut-off and annihilation operators for the Bloch modes near the band minima. The form of EFT is determined by considering lattice rotation and reflection symmetries, under which the fields φ α transform as and respectively. The Hamiltonian density of the EFT consistent with these symmetries is with effective couplings , and g ’s. At tree level, they are approximated as , and where a s is the 3D scattering length, a is the lattice constant, u Q α is the periodic Bloch wavefunction, and the integral ∫ d 3 x is over one unit cell. Details of calculation for the coupling constants are provided in the Supplementary Note 2 . Although the connection of the EFT to microscopic origins is made clear in the tree level estimate, the form of EFT resulting from symmetry analysis does not rely on this estimate. In the vicinity of thermal phase transitions of the SF phases, classical phase fluctuations are expected to dominate the universal physics, which allows us to ignore the subdominant density fluctuations and to replace φ α by with ρ the total density. In terms of phases θ α , the Hamiltonian density is rewritten as Bearing in mind the periodic nature of the phases θ α , a proper lattice regularization of this EFT leads precisely to Equation (7). How to cite this article: Li, X. et al. Proposed formation and dynamical signature of a chiral Bose liquid in an optical lattice. Nat. Commun. 5:3205 doi: 10.1038/ncomms4205 (2014).